Photocatalytic colour switching of redox dyes for ink-free light-printable rewritable paper The invention of paper as writing materials has greatly contributed to the development and spread of civilization. However, its large-scale production and usage have also brought significant environment and sustainability problems to modern society. To reduce paper production and consumption, it is highly desirable to develop alternative rewritable media that can be used multiple times. Herein we report the fabrication of a rewritable paper based on colour switching of commercial redox dyes using titanium oxide-assisted photocatalytic reactions. The resulting paper does not require additional inks and can be efficiently printed using ultraviolet light and erased by heating over 20 cycles without significant loss in contrast and resolution. The legibility of prints can retain over several days. We believe this rewritable paper represents an attractive alternative to regular paper in meeting the increasing global needs for sustainability and environmental protection. Although we now live in an age dominated by electronic media, paper still plays a very important role in communication and information storage, as evidenced by its tripled global consumption over the past three decades [1] , [2] . According to recent international surveys, 90% of all information in businesses is currently retained on paper; however, most of the prints are disposed after only one-time reading, which not only significantly increases business operating cost on both paper and ink cartridges but also creates huge environmental problems including deforestation, solid waste and chemical pollution to air, water and land [3] , [4] . Rewritable paper that can be used multiple times and does not require additional inks for printing is therefore an attractive alternative that can have enormous economical and environmental merits to modern society [5] , [6] , [7] , [8] , [9] , [10] , [11] . Conventionally, organic dyes capable of undergoing reversible colour switching based on the photoisomerization of constitute chromophores were proposed for potential use as the imaging layer in rewritable printing media [12] , [13] , [14] , [15] , [16] , [17] , [18] , [19] . However, only limited progresses have been made in this area because of some major challenges [20] , [21] , [22] : (i) colour switching often becomes much slower when dyes are present in solid media instead of solution, as their molecular mobility is markedly restricted [23] , (ii) many switchable dyes retain their colour for only several hours under ambient conditions, which is too short for reading, (iii) the toxicity of switchable dyes is often an issue for daily use and (iv) most switchable dyes involve complex synthesis and are therefore expensive. As a result, it is of high interest to develop rewritable papers based on new colour switching mechanisms [24] , [25] . Redox dyes can reversibly change colour on redox reactions. They may serve as promising imaging media for the development of rewritable paper if their redox reactions can be manipulated properly. Methylene blue (MB), for example, can be switched between blue colour in an oxidizing environment and colourless (leuco form, LMB) in a reducing environment [26] , [27] , [28] . It is a dye of low toxicity broadly used in biology and medicine, with typical applications include being an antidote for cyanide and, most commonly, in vitro diagnostic in biology, cytology, haematology and histology [29] , [30] , [31] . It has been found that TiO 2 , a photocatalytically active material, could be used to enable the decolouration of MB under UV irradiation [26] , [27] , [28] . In this case, additional reducing agents, such as ascorbic acid, were usually used as sacrificial electron donor (SED) to scavenge the holes produced from the excitation of TiO 2 under UV irradiation, and leave photo-generated electrons for reducing MB to LMB in solution. However, there is no report about using TiO 2 and MB as an imaging layer for the fabrication of light switchable rewritable paper, because the recolouration process could not be initiated by any convenient means due to the presence of excessive reducing agents in the system. TiO 2 nanocrystals capped with appropriate ligands have been recently used to promote the decolouration of an aqueous solution of MB from blue to colourless under UV irradiation, and the system can recover to its original blue colour on visible light irradiation [32] . The decolouration is mainly driven by the reduction of MB to LMB by photo-generated electrons from TiO 2 nanocrystals under UV irradiation, and the recolouration process operates by the TiO 2 -induced self-catalysed oxidation of LMB by ambient O 2 under visible irradiation. Compared with photoisomerizable chromophores, the TiO 2 /MB/water system can rapidly switch colour with high reversibility and excellent repeatability. It also has the merits of low toxicity and low cost as both TiO 2 particles and MB have already been widely used in cosmetic, medical and other industries. However, the spontaneous recolouration process under visible light makes this system incompatible with its potential use as an imaging layer in the rewritable paper. Indeed, simply depositing the solution of TiO 2 nanocrystals and MB on a solid substrate led to a flaky film, which, after decolouration by UV, can only remain colourless for <6 h, mainly due to the quick oxidation of LMB by ambient oxygen. For using as the imaging layer in the rewritable paper, a new mechanism is highly desirable to effectively stabilize the LMB and maintain the colourless state for significantly longer periods. For a redox dye-based rewritable paper, the recolouration should be slow enough to retain the printed information under ambient conditions, but sufficiently fast when external stimulation for switching is applied. In this work, we report the fabrication of a solid composite film to which letters and patterns can be repeatedly printed using UV light, retained for days and then erased by simple heating. The imaging layer of the rewritable film is composed of TiO 2 nanocrystals, a redox dye, and hydroxyethyl cellulose (HEC). This new rewritable paper can be erased and rewritten >20 times with no significant loss in resolution. In addition, rewritable paper with three primary colours (blue, red and green) can be produced by using various commercial redox dyes, such as MB, neutral red (NR) and acid green (AG). The excellent performance of these novel rewritable paper promises their potential use as an attractive alternative to a regular paper to meet our society’s increasing needs for sustainability and environmental protection. Photocatalytic colour switching In our design, the basic reactions involved in printing and erasing are the reduction and oxidation of MB. The reduction reaction is photocatalytically initiated by TiO 2 nanocrystals under UV irradiation. The TiO 2 nanocrystals with diameter of a few nanometres were synthesized through a high-temperature hydrolysis reaction in the presence of a nonionic polymeric capping ligand poly(ethylene glycol)-b-poly(propylene glycol)-b-poly(ethylene glycol) (P123), which binds to the nanocrystal surface and acts as an effective SED to scavenge holes generated from the photoexcited TiO 2 nanocrystals ( Supplementary Fig. 1 ). UV irradiation of the film therefore produces sufficient electrons for rapid reduction of blue MB to its colourless leuco form. The key challenge here is the prevention of rapid spontaneous oxidation of LMB by ambient oxygen so that the printed information can be retained legible for a reasonably long period. We choose to use HEC to address this issue, as it not only chemically stabilizes the LMB through hydrogen bonding but also reduces the diffusion of ambient oxygen ( Fig. 1 ). Adding HEC to the mixture containing TiO 2 nanocrystals and MB led to a smooth film that can retain the photoprinted mark for >3 days under ambient conditions, making the system practically useful for the fabrication of rewritable paper. 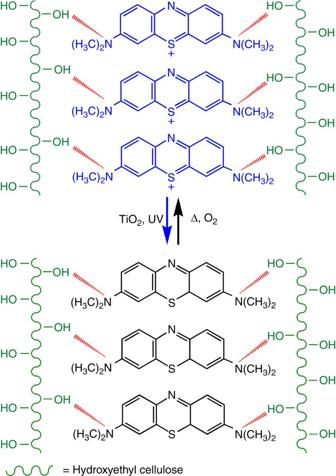Figure 1: Reversible redox reactions involved in the colour switching of a TiO2/MB/HEC composite film. MB (blue, oxidized form) and LMB (colourless, reduced form) molecules are stabilized by surrounding HEC molecules through hydrogen bonding. The chloride ion is omitted in the molecular structure of MB. Figure 1: Reversible redox reactions involved in the colour switching of a TiO 2 /MB/HEC composite film. MB (blue, oxidized form) and LMB (colourless, reduced form) molecules are stabilized by surrounding HEC molecules through hydrogen bonding. The chloride ion is omitted in the molecular structure of MB. Full size image Colour switching tests of TiO 2 /MB solid film were conducted first by directly drying TiO 2 nanocrystals/MB/water solution on a glass substrate ( Supplementary Fig. 2 ). The absorption spectrum of the solid film appeared very different from that of the aqueous mixture, in which the absorption at ~660 nm decreased while the absorption at ~590 nm increased drastically, indicating the conversion of monomers of MB to dimers (and some trimers) due to the increased MB concentration during drying. The blue coloured MB switched rapidly to colourless LMB under UV irradiation, suggesting the effective photocatalytic reduction of MB by TiO 2 nanocrystals. As expected, LMB switched back to MB completely under ambient conditions in <6 h, making the system difficult for practical applications in the rewritable paper. We found that HEC can significantly slowdown the oxidation process. The stabilization effect can be attributed to the hydrogen bonding between the abundant −OH groups on HEC molecules and the −N(CH 3 ) 2 groups on MB and LMB, as schematically shown in Fig. 1 . Our finding is supported by an earlier report by Nakata et al. [33] , although therein the interaction between HEC and MB was believed to be electrostatic. The stabilization effect can also be found even in solution, where introducing HEC to an MB solution can promote the transition of MB monomers to their dimeric form ( Supplementary Fig. 3 ), as evidenced by the progressive enhancement in the intensity of the peak at ~610 nm with increasing concentration of HEC in the solution. After mixing MB, TiO 2 nanocrystals, HEC and EG homogenously in water, the mixture remained a stable blue dispersion and no precipitation could be observed even after 3 months ( Supplementary Fig. 4 ). HEC also greatly helped with the film formation: the mixture could be conveniently drop casted on a glass or plastic substrate and produce a solid film with a homogeneous blue colour and a smooth surface, which remained unchanged in topography even after being heated to 150 °C. In addition, HEC has been widely used in cosmetics and household products as a gelling and thickening agent due to its low toxicity and cost. The introduction of HEC also helps in preventing potential exposure of human body directly to dyes, again benefiting the practical usage of the system. Reversibility and repeatability Incorporating HEC into TiO 2 /MB/HEC solid film did not show obvious effect on the decolouration rate under UV light irradiation, further indicating the effectiveness of the photoexcited TiO 2 nanocrystals in reducing MB. As shown in Fig. 2a , the absorption peak of solid film (main peak at ~660 nm) disappeared completely after 1 min of UV irradiation. However, it took 6 days to re-oxidize 20% LMB back to MB under ambient conditions, which was substantially slower than the case without HEC ( Fig. 2b ). It is therefore clear that HEC can greatly inhibit the oxidation of LMB, making the system compatible with the needs in practical applications. In contrast, although the stabilization effect of HEC is very effective at ambient conditions, heating the colourless solid film in air at 115 °C can markedly enhance the recolouration rate. As shown in Fig. 2c , when the colourless solid film containing LMB was heated in air at 115 °C, the absorption of MB monomers at ~660 nm gradually increased and fully recovered to the original intensity after 8 min. Interestingly, the heating process also indicates that monomer-to-dimer conversion is an exothermic process: after cooling in air for ~40 min, some of the MB monomers converted to dimers again with absorption peak partially shifting from ~660 to ~610 nm ( Supplementary Fig. 5 ). The reversibility and repeatability of the same solid film under two different states have been investigated. As shown in Fig. 2d , it was found that only a slight decrease in colour intensity was observed after 20 consecutive writing–erasing cycles. Throughout the 20 cycles, the TiO 2 /MB/HEC solid film remained essentially unchanged without the formation of any cracks or aggregations. It is worth noting that rewriting cycle number of 20 already represents a big step forward comparing with the existing systems [24] . We also want to point out that our systems can still operate for many more cycles beyond 20 times, although it is expected that their performance will eventually decay due to the consumption of the SED molecules. For example, by slightly increasing the amount of TiO 2 nanocrystals and simultaneously decreasing the amount of HEC in the fabrication of solid film, the cycling performance can be further enhanced to 30 cycles ( Supplementary Fig. 6 ). Note that the HEC film turned to slightly yellowish after heating at 115 °C, leading to a small increase in the intensity of the background absorption. 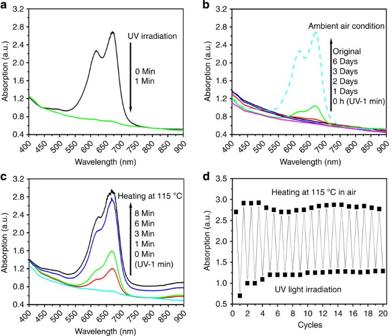Figure 2: Reversible colour switching of the TiO2/MB/HEC solid film. (a) UV–vis spectra showing the decolouration process under UV irradiation; (b) UV–vis spectra showing the recolouration of the film at room temperature under ambient air; (c) UV–vis spectra showing the recolouration process on heating at 115 °C in air and (d) the absorption intensity of a solid film recorded continuously in 20 cycles of switching between colour and colourless states. The HEC film turned to slightly yellow on heating at 115 °C, and therefore increased the intensity of the background absorption. Figure 2: Reversible colour switching of the TiO 2 /MB/HEC solid film. ( a ) UV–vis spectra showing the decolouration process under UV irradiation; ( b ) UV–vis spectra showing the recolouration of the film at room temperature under ambient air; ( c ) UV–vis spectra showing the recolouration process on heating at 115 °C in air and ( d ) the absorption intensity of a solid film recorded continuously in 20 cycles of switching between colour and colourless states. The HEC film turned to slightly yellow on heating at 115 °C, and therefore increased the intensity of the background absorption. Full size image Controlling the recolouration rate We have also explored the effect of HEC concentration on the stability of LMB under ambient conditions. As shown in Fig. 3 , it was clear that the recolouration process became significantly slower when the concentration of HEC increased in the solid film. In addition to its chemical stabilization effect on LMB, HEC may also contribute to the enhanced stability by partially blocking the diffusion of O 2 to LMB through the film. When the concentration of HEC was reduced to half from the case in Fig. 2 , the decolouration by UV irradiation can still complete quickly within 1 min ( Supplementary Fig. 7a ). However, recolouration of the film under ambient conditions became faster, and the film colour completely recovered after ~36 h sitting in air ( Fig. 3b and Supplementary Fig. 7b ). Consistently, the heating temperature required for recolouration can be reduced to 90 °C: only 5 min was needed for complete recolouration when heated in air at this temperature ( Supplementary Fig. 7c ). As indicated in Fig. 3c , when the TiO 2 /MB/HEC film is overcoated with an additional layer of pure HEC, the recolouration can slowdown considerably. 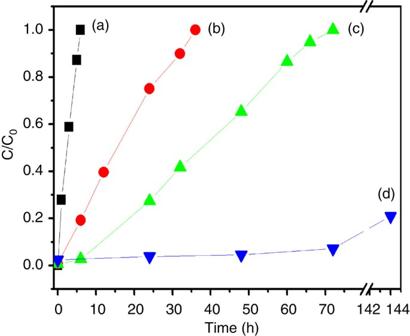Figure 3: The effect of HEC on recolouration rate. Plots of the percent of MB recovered from LMB in solid films by monitoring the absorbance of MB after UV light irradiation as a function of time in ambient air: (a) TiO2nanocrystals/MB, (b) TiO2nanocrystals/MB/HEC, (c) TiO2nanocrystals/MB/HEC with additional HEC film on top surface and (d) TiO2nanocrystals/MB/HEC solid film with concentration of HEC doubled from the case in (b). When calculating C/C0, the contribution of HEC to the absorption background was subtracted for all samples. Figure 3: The effect of HEC on recolouration rate. Plots of the percent of MB recovered from LMB in solid films by monitoring the absorbance of MB after UV light irradiation as a function of time in ambient air: (a) TiO 2 nanocrystals/MB, (b) TiO 2 nanocrystals/MB/HEC, (c) TiO 2 nanocrystals/MB/HEC with additional HEC film on top surface and (d) TiO 2 nanocrystals/MB/HEC solid film with concentration of HEC doubled from the case in (b). When calculating C/C 0 , the contribution of HEC to the absorption background was subtracted for all samples. Full size image High-resolution photo-printing The excellent reversibility and repeatability make the TiO 2 /MB/HEC composite film ideal for use as a rewritable paper. As a demonstration, we printed letters and patterns in the film by UV light irradiation through a photomask, which was pre-produced by ink-jet printing on a plastic transparency ( Fig. 4a ). After UV irradiation for ~2 min, the exposed regions turned to white, whereas the unexposed regions retained the blue colour, replicating letters/patterns from the photomask to the film, as shown in Fig. 4b . One of the advantages of the system is the convenience in producing a large-scale film. To demonstrate the practical application, we have printed a paragraph of letters on a 5 × 6.5 cm 2 film. As shown in Fig. 4c , blue letters of font size 10 with very good resolution could be easily achieved, and they remained highly legible for at least 3 days under ambient conditions ( Fig. 4d,e ), which is sufficiently long for most of the temporary reading purposes. In fact, the printed letters were still readable even after 5 days ( Fig. 4f ), although the background gradually turned to light blue. The contrast of the letters started to show apparent decay after 8 days ( Supplementary Fig. 8 ). The prints can be erased completely by heating the rewritable paper at 115 °C in air for ~10 min. The slight variation in the background of the printed images was due to the uneven thickness of the film resulted from the manual drop casting. This issue could be resolved by making more uniform films after some practice ( Supplementary Fig. 9 ) or by employing more automated processes. In addition, various complicated patterns can also be printed on the rewritable paper with excellent resolution, as shown in the examples in Fig. 5 , which were produced after >10 consecutive writing–erasing cycles. No decrease in colour intensity and resolution of the written patterns was observed. In addition to glass substrates, the composite film can also be deposited on plastic substrates and produce a flexible rewritable paper ( Supplementary Fig. 10 ). To demonstrate the high-resolution printing achievable in our rewritable paper, we have printed microscale patterns through a chrome photomask ( Supplementary Fig. 11 ) using again a commercial UV lamp. As shown in the optical microscopy images in Fig. 6 , various microscale patterns with sizes from 550 to 35 μm could be successfully photoprinted on the rewritable film. Compared with the patterns on the original photomask, the sharp edges of the photo-printed microscale patterns clearly demonstrate the high resolution achievable in this system. 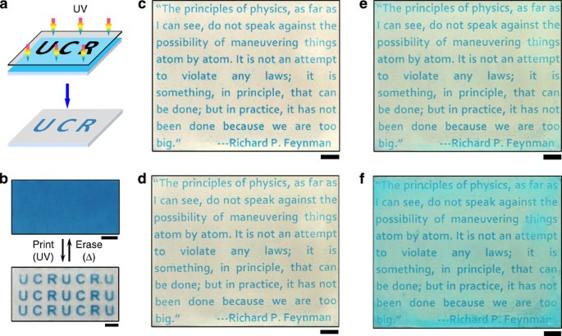Figure 4: Printing, erasing and legibility of letters on the rewritable paper. (a) Schematic representation of writing letters on the rewritable paper using photomask on UV light irradiation, (b) digital images of writing and erasing letters on the rewritable paper, (c–f) digital images of rewritable paper maintaining in ambient air after writing of (c) 10 min, (d) 1 day, (e) 3 days and (f) 5 days. Scale bars, 5 mm. The photomask was produced by ink-jet printing on a plastic transparency. The slight variation in the background was due to the uneven thickness of the film resulted from the manual drop casting. Figure 4: Printing, erasing and legibility of letters on the rewritable paper. ( a ) Schematic representation of writing letters on the rewritable paper using photomask on UV light irradiation, ( b ) digital images of writing and erasing letters on the rewritable paper, ( c – f ) digital images of rewritable paper maintaining in ambient air after writing of ( c ) 10 min, ( d ) 1 day, ( e ) 3 days and ( f ) 5 days. Scale bars, 5 mm. The photomask was produced by ink-jet printing on a plastic transparency. The slight variation in the background was due to the uneven thickness of the film resulted from the manual drop casting. 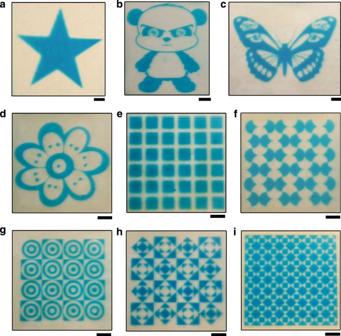Figure 5: Printing complex patterns on the rewritable paper. The prints were produced after >10 consecutive writing–erasing cycles. Scale bar, 5 mm. Full size image Figure 5: Printing complex patterns on the rewritable paper. The prints were produced after >10 consecutive writing–erasing cycles. Scale bar, 5 mm. 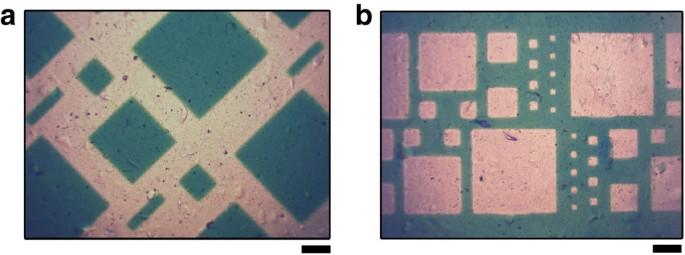Figure 6: Optical microscopy images of photo-printed microscale patterns. The microscale patterns were photoprinted on a rewritable film using a laboratory 365-nm UV lamp through a chrome photomask. The sharp edges of the microscale patterns demonstrate high-resolution printing. Scale bar, 200 μm. Full size image Figure 6: Optical microscopy images of photo-printed microscale patterns. The microscale patterns were photoprinted on a rewritable film using a laboratory 365-nm UV lamp through a chrome photomask. The sharp edges of the microscale patterns demonstrate high-resolution printing. Scale bar, 200 μm. Full size image Photo-printing with multiple coloured dyes The design principle described in this work allows us to change the working colours of rewritable paper by replacing MB with other commercial redox dyes. For example, replacing MB with NR produced a film that can be reversibly switched from red to colourless after UV exposure. Introducing AG to the composite film led to a rewritable paper that can switch from green to light yellow by UV irradiation. 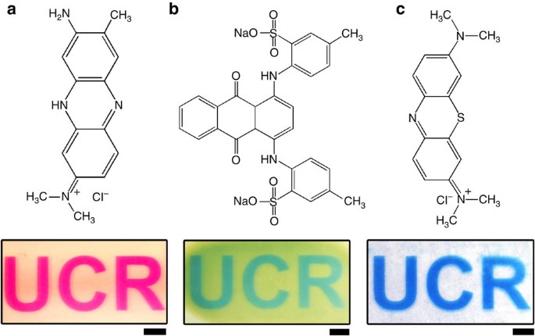Figure 7: Letters photoprinted with RGB colours. The rewritable composite films were fabricated by using (a) neutral red, (b) acid green and (c) methylene blue. Scale bars, 5 mm. Figure 7 demonstrates the red, green and blue coloured letters photoprinted on films containing the three different dyes. We believe a more complete survey of the redox dyes for incorporation into our system would provide more options of working colours for the rewritable paper. Figure 7: Letters photoprinted with RGB colours. The rewritable composite films were fabricated by using ( a ) neutral red, ( b ) acid green and ( c ) methylene blue. Scale bars, 5 mm. Full size image We have demonstrated here an effective and economic strategy for the development of a new type of rewritable paper, in which a commercial redox dye is introduced as the imaging layer. While printing is achieved by photobleaching the dye through UV irradiation with TiO 2 nanocrystals as catalysts, erasing is initiated by heating, which significantly promotes the recolouration process through oxidation of the dye by ambient oxygen. The problem of fast recolouration under ambient conditions could be addressed by adding HEC to the system, which not only stabilizes the reduced dye through hydrogen bonding but also blocks oxygen diffusion to the dye. More than 20 printing–erasing cycles have been realized without observable colour fading, and the printed letters remain legible with high resolution at ambient conditions for > 3 days, which is long enough for many practical applications involving temporary reading such as newspapers. Furthermore, our rewritable paper has advantages over the previously reported versions of rewritable media, including simple paper making process, low production cost, low toxicity and low energy consumption. Our rewritable paper is an attractive alternative to a regular paper to address the increasing problems in environment and resource sustainability. The design principle can be extended to various commercial redox dyes to produce a rewritable paper capable of showing prints of different colours. It is believed that more elaborate features, such as multicolour printing on the same page, may be realized in the future with further advancement in controlling the redox reactions of the dyes, for example, by selective photoreduction of the dyes by lights of different wavelengths. Chemicals Titanium (IV) chloride (TiCl 4 ), diethylene glycol (DEG), ethylene glycol (EG), poly(ethylene glycol)-b-poly(propylene glycol)-b-poly(ethylene glycol) (P123), ammonium hydroxide (NH 4 OH),HEC, MB, NR and AG were purchased from Sigma-Aldrich. All other chemical reagents were of analytical grade and used as received without further purification. Characterization The absorption spectra of the solid film were measured by a UV–vis spectrophotometer (HR2000CG-UV-NIR, Ocean Optics). The morphology of the nanostructures was investigated using a Philips Tecnai T12 transmission electron microscope at an accelerating voltage of 120 kV. Microscale patterns photoprinted on the rewritable paper were imaged in transmission mode using an Omano OM339P optical microscope. Synthesis of TiO 2 nanocrystals TiO 2 nanocrystals were synthesized using a high-temperature hydrolysis reaction reported previously [32] . Typically, a mixture containing TiCl 4 (1 ml), P123 (0.6 g), NH 4 OH (1 ml), and DEG (20 ml) in a 100-ml flask was heated to ~220 °C in air under vigorous stirring, forming a transparent solution. The resulting mixture was kept at 220 °C for 3 h and then cooled to room temperature. A light-brown mud-like precipitate was obtained on adding acetone and centrifuging at 11,000 r.p.m. for 10 min. The product was washed several times with ethanol and acetone to remove residuals, and then redispersed in water at concentrations of 10 or 20 mg ml −1 . A typical TEM image of the TiO 2 nanocrystals is shown in Supplementary Fig. 1 . Preparation of solid film An HEC/H 2 O stock solution was prepared by dissolving HEC (1.0 g) in H 2 O (30 ml) at 65 °C. Typically, TiO 2 /H 2 O dispersion (20 mg ml −1 , 4 ml), MB/H 2 O solution (0.01 M, 800 μl), HEC/H 2 O stock solution (4 ml) and EG (1 ml) were mixed together and sonicated to form a homogenous solution. The solution (~2.5 ml) was drop casted directly on a glass or plastic substrate (50 × 65 mm 2 ) and then dried in an oven at 80 °C for 12 h to form a solid blue film. Including a small amount of EG to the mixture solution could improve the smoothness of the solid film. For making a solid film with half concentration of HEC than typical case, a mixture of HEC/H 2 O stock solution (1 ml), TiO 2 /H 2 O dispersion (10 mg ml −1 , 4 ml), MB/H 2 O solution (0.01 M, 400 μl), H 2 O (3 ml) and EG (1 ml) was used. In a control experiment, a mixture of HEC/H 2 O stock solution (1 ml), EG (1 ml) and H 2 O (5 ml) was drop casted on top of the solid composite film to form an additional HEC layer. Photoirradiation Photoirradiation was performed using a typical laboratory 365-nm UV lamp. How to cite this article: Wang, W. et al. Photocatalytic colour switching of redox dyes for ink-free light-printable rewritable paper. Nat. Commun. 5:5459 doi: 10.1038/ncomms6459 (2014).